Modest CaV1.342-selective inhibition by compound8is β-subunit dependent Two voltage-gated calcium channel subtypes—Ca V 1.2 and Ca V 1.3—underlie the major L-type Ca 2+ currents in the mammalian central nervous system. Owing to their high sequence homology, the two channel subtypes share similar pharmacological properties, and at high doses classic calcium channel blockers, such as dihydropyridines, phenylalkylamines and benzothiazepines, do not discriminate between the two channel subtypes. Recent progress in treating Parkinson’s disease (PD) was marked by the discovery of synthetic compound 8 , which was reported to be a highly selective inhibitor of the Ca V 1.3 L-type calcium channels (LTCC). However, despite a previously reported IC 50 of ~24 μM, in our hands inhibition of the full-length Ca V 1.3 42 by compound 8 at 50 μM reaches a maximum of 45%. Moreover, we find that the selectivity of compound 8 towards Ca V 1.3 relative to Ca V 1.2 B15 channels is greatly influenced by the β-subunit type and its splice isoform variants. Parkinson’s disease (PD) is a movement disorder arising from the degeneration of dopaminergic neurons in the substantia nigra pars compacta (SNc). Although mutations of several genes have been associated with PD [1] , 95% of PD cases are idiopathic. The over-reliance of Ca V 1.3 current for pacemaking in the adult SNc neurons was reported to aggravate mitochondrial oxidative stress [2] , and consequently enhance the susceptibility of these neurons towards toxins such as MPTP (1-methyl-4-phenyl-1,2,3,6-tetrahydropyridine) and rotenone [3] . Significantly, pharmacological blockade or genetic deletion of Ca V 1.3 channels confers protection against toxin induced neuronal damage [3] . Interestingly, population studies also revealed significant reduction in the risk of developing PD among hypertensive subjects receiving dihydropyridines (DHPs), classical blockers of L-type calcium channels [4] , [5] . Voltage-gated calcium channels Ca V 1.2 and Ca V 1.3 underlie the majority of L-type calcium currents in the central nervous system. While Ca V 1.3 channels contribute only 20% of the total L-type currents in the central nervous system, the use of non-selective DHPs that also inhibits Ca V 1.2 channels could have profound neuro-physiological consequences [6] . In addition, neuronal transcripts of Ca V 1.3 channels display extensive alternative splicing patterns, generating splice variants with different biophysical and pharmacological properties [7] , [8] , [9] . The Ca V 1.3 42a splice variant with a truncated C terminus displayed attenuated sensitivity towards DHP as compared with the long-form Ca V 1.3 42 channels [8] . Tissue-selective expression of various Ca V 1.3 splice variants would therefore require different dosages for effective inhibition of the Ca V 1.3 currents. Recently, Kang et al. [10] reported the identification of 1-(3-chlorophenethyl)-3-cyclopentylpyrimidine-2,4,6(1H,3H,5H)-trione, also known as compound 8 as a pharmacological blocker highly selective for Ca V 1.3 (IC 50 =24.3±0.7 μM) over Ca V 1.2 channels. In the current study, we evaluated compound 8 for its activity against different Ca V 1.3 channel splice isoforms. Unexpectedly, initial heterologous expression in human embryonic kidney 293 (HEK293) cells co-transfected with β2a-subunit revealed that compound 8 inhibited Ca V 1.2 more than either Ca V 1.3 42 or Ca V 1.3 42a channels. Replacing β2a-subunit with β1-, β3- or β4-subunit on the other hand yielded results that showed modest selective inhibition of compound 8 against Ca V 1.3 42 over Ca V 1.2 B15 channels. However, there was clearly no selective inhibition of compound 8 against Ca V 1.3 42a and Ca V 1.2 channels in the presence of anyone of the other three β-subunits. Based on the existing data, we conclude that the Ca V 1.3-selective inhibition by compound 8 is modest and is highly dependent on the composition of the Ca V 1.3 splice variant in association with a particular type of β-subunit. Compound 8 is not selective against Ca V 1.3 with β 2a-subunit Compounds 1 , 8 and PYT (1,3-bis(4-chlorophenethyl)pyrimidine-2,4,6(1H, 3H, 5H)-trione; Fig. 1 ) were synthesized according to the procedure reported by Kang. et al. [10] but with slight modifications (see Methods section). It has been reported that the newly discovered compound 8 inhibited ~30 and 60% of Ca V 1.3 current at concentrations of 5 and 50 μM, respectively, whereas Ca V 1.2 channels were weakly responsive as 50 μM of compound 8 inhibited only close to 10% of its peak current [10] . 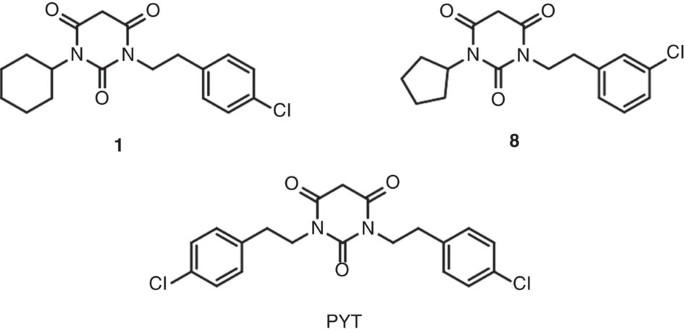Figure 1 Structures of compounds1,8andPYT. Figure 1 Structures of compounds 1 , 8 and PYT . Full size image We have recently discovered that alternative splicing at the C terminus regulated the sensitivity of Ca V 1.3 channels towards DHPs; while the long-form Ca V 1.3 42 channel exhibited high sensitivity towards DHP; truncation of the C terminus immediately after the IQ domain via alternate use of exon 42a yielded the less sensitive Ca V 1.3 42a channel [8] . To determine whether the compound 8 may also have differential effects on different C-terminal splice forms, we first tested the sensitivity of rat Ca V 1.3 42 and Ca V 1.3 42a . In the presence of β2a contransfected with the Ca V 1.3 channels, the channel isoforms displayed very little run-down with repeated 1 s square pulse depolarization to test potential of 10 mV from a holding potential of −70 mV at the frequency of 0.05 Hz ( Figs 2b and 3b ). Surprisingly, 5 μM of compound 8 failed to significantly inhibit the peak Ca 2+ current ( I Ca ) of either Ca V 1.3 42 or Ca V 1.3 42a ( Figs 2 and 3 ) as compared with the untreated controls. Moreover, 50 μM of compound 8 only inhibited 29.51±3.01 and 23.57±2.14% of the peak I Ca of Ca V 1.3 42 or Ca V 1.3 42a , respectively ( Figs 2 and 3 ). In addition, Ca V 1.3 42 channels were blocked to a similar level with compound 8 obtained from an additional source ( Supplementary Fig. 1 ). In comparison, 78.85±2.63% of Ca V 1.3 42 current and 68.14±3.43% of Ca V 1.3 42a current could be robustly inhibited by 5 μM of nimodipine ( Figs 2 and 3 ). As compound 8 has been reported to have little effect on Ca V 1.2 current, we tested its inhibition on the rat Ca V 1.2 B15 channels [11] . As compared with the Ca V 1.3, a slightly enhanced run-down effect (10.14±3.98%) was observed for Ca V 1.2 B15 channels ( Fig. 4b ). However, 34.97±4.39 and 44.03±4.67% of Ca V 1.2 B15 current could be inhibited by 5 and 50 μM of compound 8 , respectively, indicating a stronger inhibitory effect of compound 8 on Ca V 1.2 than Ca V 1.3 channels. As expected, 80.66±2.82% of Ca V 1.2 B15 current was blocked by 5 μM nimodipine ( Fig. 4 ). 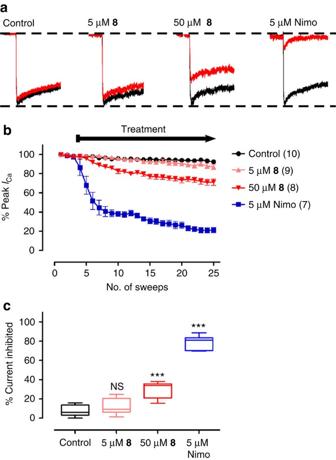Figure 2: Inhibition of CaV1.342current by compound8and nimodipine (Nimo). (a) Representative traces of CaV1.342currents recorded by single 1 s square pulse to test potential of 10 mV from holding potential of −70 mV for 25 sweeps with sweep interval of 20 s. Only the first three untreated (black) and last three treated (red) traces are shown for each treatment groups. Displayed are the first 100 ms of each recording trace. (b) Averaged diary plot of effects of either control, 5 μM8, 50 μM8or 5 μM Nimo on CaV1.342peak currents. The number of cells analysed are indicated in the parenthesis. The drugs were added after the three stable sweeps. (c) Population data of the % peak current inhibition at the 25th sweep normalized against the first sweep conferred by either 5 μM8, 50 μM8or 5 μM Nimo as compared with the control. NS, non-significant. ***P<0.001 (Student’s unpairedt-test). Alternatively,P<0.001 among all the treatment groups (one-way analysis of variance and Bonferroni’s test). The number of cells analysed is indicated inb. The data for each condition were collected from two to three transfections. Figure 2: Inhibition of Ca V 1.3 42 current by compound 8 and nimodipine (Nimo). ( a ) Representative traces of Ca V 1.3 42 currents recorded by single 1 s square pulse to test potential of 10 mV from holding potential of −70 mV for 25 sweeps with sweep interval of 20 s. Only the first three untreated (black) and last three treated (red) traces are shown for each treatment groups. Displayed are the first 100 ms of each recording trace. ( b ) Averaged diary plot of effects of either control, 5 μM 8 , 50 μM 8 or 5 μM Nimo on Ca V 1.3 42 peak currents. The number of cells analysed are indicated in the parenthesis. The drugs were added after the three stable sweeps. ( c ) Population data of the % peak current inhibition at the 25th sweep normalized against the first sweep conferred by either 5 μM 8 , 50 μM 8 or 5 μM Nimo as compared with the control. NS, non-significant. *** P <0.001 (Student’s unpaired t -test). Alternatively, P <0.001 among all the treatment groups (one-way analysis of variance and Bonferroni’s test). The number of cells analysed is indicated in b . The data for each condition were collected from two to three transfections. 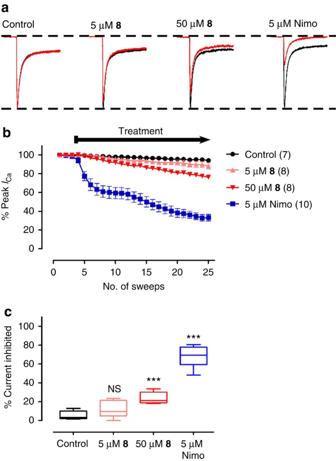Figure 3: Inhibition of CaV1.342acurrent by compound8and nimodipine (Nimo). (a) Representative traces of CaV1.342acurrents, format as inFig. 2a. (b) Averaged diary plot of effects either control, 5 μM8, 50 μM8or 5 μM Nimo on CaV1.342apeak currents, format as inFig. 2b. (c) Population data of the % peak current inhibition at the 25th sweep normalized against the first sweep conferred by either 5 μM8, 50 μM8or 5 μM Nimo as compared with the control. NS, non-significant. ***P<0.001 (Student’s unpairedt-test). Alternatively,P<0.001 among all the treatment groups (one-way analysis of variance and Bonferroni’s test). The number of cells analysed is indicated inb. The data for each condition were collected from two to three transfections. Full size image Figure 3: Inhibition of Ca V 1.3 42a current by compound 8 and nimodipine (Nimo). ( a ) Representative traces of Ca V 1.3 42a currents, format as in Fig. 2a . ( b ) Averaged diary plot of effects either control, 5 μM 8 , 50 μM 8 or 5 μM Nimo on Ca V 1.3 42a peak currents, format as in Fig. 2b . ( c ) Population data of the % peak current inhibition at the 25th sweep normalized against the first sweep conferred by either 5 μM 8 , 50 μM 8 or 5 μM Nimo as compared with the control. NS, non-significant. *** P <0.001 (Student’s unpaired t -test). Alternatively, P <0.001 among all the treatment groups (one-way analysis of variance and Bonferroni’s test). The number of cells analysed is indicated in b . The data for each condition were collected from two to three transfections. 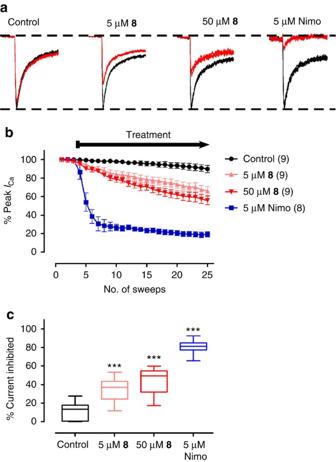Figure 4: Inhibition of CaV1.2B15current by compound8and nimodipine (Nimo). (a) Representative traces of CaV1.2B15currents, format as inFig. 2a. (b) Averaged diary plot of effects of either control, 5 μM8, 50 μM8or 5 μM Nimo on CaV1.2B15peak currents, format as inFig. 2b. (c) Population data of the % peak current inhibition at the 25th sweep normalized against the first sweep conferred by either 5 μM8, 50 μM8or 5 μM Nimo as compared with the control. ***P<0.001. (Student’s unpairedt-test) Alternatively,P<0.001 among all the treatment groups (one-way analysis of variance and Bonferroni’s test). The number of cells analysed is indicated inb. The data for each condition were collected from two to three transfections. Full size image Figure 4: Inhibition of Ca V 1.2 B15 current by compound 8 and nimodipine (Nimo). ( a ) Representative traces of Ca V 1.2 B15 currents, format as in Fig. 2a . ( b ) Averaged diary plot of effects of either control, 5 μM 8 , 50 μM 8 or 5 μM Nimo on Ca V 1.2 B15 peak currents, format as in Fig. 2b . ( c ) Population data of the % peak current inhibition at the 25th sweep normalized against the first sweep conferred by either 5 μM 8 , 50 μM 8 or 5 μM Nimo as compared with the control. *** P <0.001. (Student’s unpaired t -test) Alternatively, P <0.001 among all the treatment groups (one-way analysis of variance and Bonferroni’s test). The number of cells analysed is indicated in b . The data for each condition were collected from two to three transfections. Full size image In addition, we evaluated the inhibitory activities of PYT and compound 1 against Ca V 1.3 and Ca V 1.2 channels [10] . Kang et al. [10] reported that PYT was the original scaffold that displayed an eightfold selectivity for Ca V 1.3, whereas compound 1 was one of the PYT analogues that was 28 times more selective for Ca V 1.3 channels. However, in our experiments, 5 μM of PYT and compound 1 did not significantly inhibit the peak I Ca of Ca V 1.3 42 ( Supplementary Fig. 2 ). In addition, 5 μM of PYT inhibited 19.90±2.59% of Ca V 1.3 42a current, whereas 5 μM of compound 1 had no effect on Ca V 1.3 42a channels ( Supplementary Fig. 3 ). In comparison, PYT and compound 1 also appeared to be more selective for Ca V 1.2 B15 showing 43.52±4.83% and 31.69±4.83% inhibition, respectively, ( Supplementary Fig. 4 ). The effect could not be a result of current run-down as little current decay was observed for the untreated Ca V 1.2 current upon prolonged pulses, and the current density of the recorded cells under all treatment groups were not significantly different in the study ( Supplementary Fig. 5 ). Furthermore, we noted that the use of the original rat Ca V 1.3 42 (ref. 12 ) (Genbank accession no. AF370010) by Kang et al. [10] contained three mutations, including G244S, A1104V and V2123A, that have been shown to drastically alter both the biophysical and pharmacological properties of the channel [9] , [13] , [14] . To test whether the use of uncorrected Ca V 1.3 42 channel, named here as Ca V 1.3 42_UC , could account for the lack of selectivity of compound 8 against Ca V 1.3 channels in the presence of β2a-subunit, we measured the sensitivity of Ca V 1.3 42_UC to either 5 and 50 μM compound 8 or 5 μM nimodipine with instead shorter 100 ms depolarizing pulse that was used by Kang et al. [10] While 5 μM compound 8 has little effect on Ca V 1.3 42_UC channels as compared with control treatment, only 15.75±3.25% of the peak current could be inhibited by 50 μM compound 8, and expectedly 73.10±3.48% of the current was blocked by 5 μM nimodipine ( Fig. 5 ). Hence, it was consistent that in the presence of β2a-subunit, Ca V 1.2 displayed higher sensitivity to compound 8 as compared with Ca V 1.3 channels. 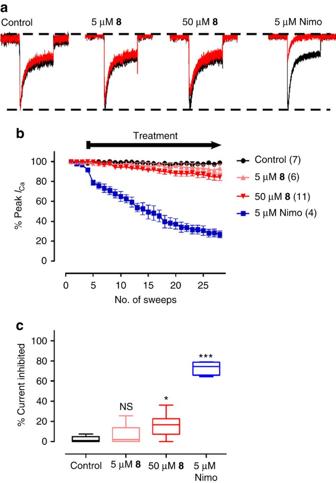Figure 5: Inhibition of CaV1.342_UCcurrent by compound8and nimodipine (Nimo). (a) Representative traces of uncorrected CaV1.242_UCcurrents, format as inFig. 2a. The current was recorded by single square pulse from holding of −70 to 10 mV for over 100 ms with sweep interval of 20 s. (b) Averaged diary plot of effects of either control, 5 μM8, 50 μM8or 5 μM Nimo on CaV1.342_UCpeak currents, format as inFig. 2b. (c) Population data of the % peak current inhibition at the 28th sweep normalized against the first sweep conferred by either 5 μM8, 50 μM8or 5 μM Nimo as compared with the control. *P<0.05, ***P<0.001 (Student’s unpairedt-test). Alternatively,P<0.001 among all the treatment groups (one-way analysis of variance and Bonferroni’s test). The number of cells analysed is indicated inb. The data for each condition were collected from two to three transfections. Figure 5: Inhibition of Ca V 1.3 42_UC current by compound 8 and nimodipine (Nimo). ( a ) Representative traces of uncorrected Ca V 1.2 42_UC currents, format as in Fig. 2a . The current was recorded by single square pulse from holding of −70 to 10 mV for over 100 ms with sweep interval of 20 s. ( b ) Averaged diary plot of effects of either control, 5 μM 8 , 50 μM 8 or 5 μM Nimo on Ca V 1.3 42_UC peak currents, format as in Fig. 2b . ( c ) Population data of the % peak current inhibition at the 28th sweep normalized against the first sweep conferred by either 5 μM 8 , 50 μM 8 or 5 μM Nimo as compared with the control. * P <0.05, *** P <0.001 (Student’s unpaired t -test). Alternatively, P <0.001 among all the treatment groups (one-way analysis of variance and Bonferroni’s test). The number of cells analysed is indicated in b . The data for each condition were collected from two to three transfections. Full size image β-subunit influences compound 8 selectivity Although it has been shown that the presence of different β-subunits did not overtly affect the sensitivity of L-type channels towards DHP [15] , the use of different β-subunits such as β3 in Kang et al. [10] and β2a in the current study might account for the opposite selectivity of compound 8 on Ca V 1.2 and Ca V 1.3 channels observed in these two studies. To test this possibility, we first measured the effect of 50 μM compound 8 on Ca V 1.3 42 , Ca V 1.3 42_UC , Ca V 1.2 B15 and Ca V 1.3 42a channels co-transfected with β3-subunit. Interestingly, while ~40% of the peak I Ca of Ca V 1.3 42 and the uncorrected Ca V 1.3 42_UC were similarly inhibited by 50 μM compound 8 , Ca V 1.2 B15 and Ca V 1.3 42a channels displayed a slightly but significantly weaker sensitivity in comparison with Ca V 1.3 42 channels as 23.47±2.60 and 29.05±2.48% of respective peak currents were inhibited ( Fig. 6 and Supplementary Fig. 6 ). Additional experiments done using either β1- and β4-subunits produced results that demonstrated enhanced inhibitory effect of compound 8 on Ca V 1.3 42 as compared with Ca V 1.3 42_UC , Ca V 1.2 B15 and Ca V 1.3 42a channels. However, Ca V 1.2 B15 and Ca V 1.3 42a channels were inhibited to similar level by 50 μM compound 8 in the presence of β1-, β3- and β4-subunits ( Fig. 6 and Supplementary Fig. 6 ). Significantly, in the presence of β2a, Ca V 1.2 B15 still displayed higher sensitivity as compared with Ca V 1.3 42 , Ca V 1.3 42_UC and Ca V 1.3 42a , even when the currents were repeatedly recorded with a shorter100-ms depolarizing square pulse ( Fig. 6 and Supplementary Fig. 6 ). Finally, we performed analysis of the correlation of the % of inhibition with the current density for each of the Ca V 1.3 42 , Ca V 1.3 42_UC , Ca V 1.2 B15 , and Ca V 1.3 42a channels. Only weak correlations were observed as indicated by the following R 2 values: 0.0121 for Ca V 1.3 42 , 0.0859 for Ca V 1.3 42_UC , 0.2439 for Ca V 1.2 B15 and 0.2047 for Ca V 1.3 42a . Therefore, the inhibitory effect of compound 8 on the Ca V 1.2 and Ca V 1.3 channels are not influenced by the amplitudes of the currents. ( Supplementary Fig. 7 ). 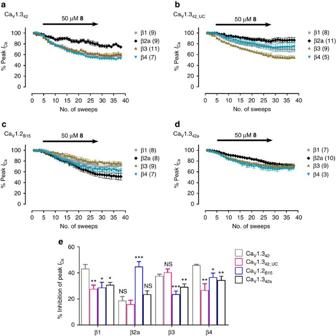Figure 6: Inhibition of CaV1.342, CaV1.342_UC, CaV1.2B15and CaV1.342acurrent by 50 μM compound8in the presence of differentβ-subunits. (a) Averaged diary plot of effects of 50 μM 8 on CaV1.342peak currents in the presence ofβ1-,β2a-,β3- and β4-subunit. The current was recorded by single square pulse from holding of −70 to 10 mV for over 100 ms with sweep interval of 20 s. (b–d) Averaged diary plot of effects of 50 μM8on the peak currents of CaV1.342_UC, CaV1.2B15and CaV1.342a, respectively, in the presence of different β-subunits, format as ina. (e) Comparison of the % peak current inhibition at the 28th sweep normalized against the first sweep conferred by 50 μM8for CaV1.342, CaV1.342_UC, CaV1.2B15, CaV1.342ain the presence of different β-subunits. Within each β-subunit, the % inhibitions of CaV1.342_UC, CaV1.2B15, CaV1.342awere compared with that of CaV1.342. NS, non-significant, *P<0.05, **P<0.01, ***P<0.001 (Student’s unpairedt-test). Alternatively,P<0.001 within each group (one-way analysis of variance and Bonferroni’s test). The number of cells analysed is indicated inb–d. The data for each condition were collected from two to three transfections. Figure 6: Inhibition of Ca V 1.3 42 , Ca V 1.3 42_UC , Ca V 1.2 B15 and Ca V 1.3 42a current by 50 μM compound 8 in the presence of different β -subunits. ( a ) Averaged diary plot of effects of 50 μM 8 on Ca V 1.3 42 peak currents in the presence of β 1-, β 2a-, β 3- and β4-subunit. The current was recorded by single square pulse from holding of −70 to 10 mV for over 100 ms with sweep interval of 20 s. ( b – d ) Averaged diary plot of effects of 50 μM 8 on the peak currents of Ca V 1.3 42_UC , Ca V 1.2 B15 and Ca V 1.3 42a , respectively, in the presence of different β-subunits, format as in a . ( e ) Comparison of the % peak current inhibition at the 28th sweep normalized against the first sweep conferred by 50 μM 8 for Ca V 1.3 42 , Ca V 1.3 42_UC , Ca V 1.2 B15 , Ca V 1.3 42a in the presence of different β-subunits. Within each β-subunit, the % inhibitions of Ca V 1.3 42_UC , Ca V 1.2 B15 , Ca V 1.3 42a were compared with that of Ca V 1.3 42 . NS, non-significant, * P <0.05, ** P <0.01, *** P <0.001 (Student’s unpaired t -test). Alternatively, P <0.001 within each group (one-way analysis of variance and Bonferroni’s test). The number of cells analysed is indicated in b – d . The data for each condition were collected from two to three transfections. Full size image PD is a debilitating movement disorder currently with no cure. The constant Ca 2+ influx via the Ca V 1.3 channels enhances mitochondrial oxidative stress that could contribute towards the pathogenesis of PD. The presence of other possible pacemaking current underlied by hyperpolarization-activated and cyclic nucleotide-gated cation (HCN) channel suggested that it might be feasible to block Ca V 1.3 current without grossly affecting the normal physiological functions of SNc neurons [3] . The availability of a Ca V 1.3 channel-specific antagonist that could eventually replace non-selective L-type blockers such as DHPs would therefore be ideal for the therapeutic management of PD. In contrast to the IC 50 of 24.3 ±0.7 μM as determined using patch-clamp electrophysiology by Kang et al. [10] , our initial data with β2a-subunits revealed that the percentage inhibition of compound 8 on Ca v 1.3 channels at 50 μM was only 30% while at 5 μM no significant inhibition was observed. In contrast to the published report, the inhibition of Ca v 1.2 channels at 50 and 5 μM were 44% and 35%, respectively, indicating selectivity of compound 8 against Ca v 1.2 channels. The initial failure to observe any selectivity of compound 8 in inhibiting Ca V 1.3 channels led us to investigate the effect of compound 8 with other β-subunits. However, while the Ca V 1.3 42 current was indeed more sensitive than Ca v 1.2 in the presence of β1-, β3- and β4-subunits, only 35–45% of the its peak currents could be blocked by 50 μM compound 8 , and the percentage of inhibition on Ca V 1.2 B15 channels was a modest 10–15% less as compared with Ca V 1.3 42 channels. To complicate the story further, the short-form Ca V 1.3 42a channels displayed similar level of sensitivity as compared with Ca V 1.2 B15 channels with either β1-, β3- or β4-subunit co-transfected. The Ca V 1.3 42a splice variant accounts for ~30% of the total Ca V 1.3 transcripts in the substantial nigra region [7] . While the roles of different Ca V 1.3 splice variants in neurodegeneration of SNc neurons in the pathogenesis of PD awaits further clarification, the larger current density and more hyperpolarized-shifted I-V relationship implied a greater involvement of Ca V 1.3 42a current in driving the pacemaking acitivity in the SNc neurons as compared with the full-length Ca V 1.3 42 channels [8] . In summary, the newly reported compound 8 is not a potent blocker of Ca V 1.3 channels as compared with the classical L-type blockers such as the DHPs. The selectivity of compound 8 on Ca V 1.3 42 over Ca V 1.2 B15 channels could be influenced strongly by the presence of various β-subunits and the compound 8 was not selective for Ca V 1.3 42a over Ca V 1.2 B15 channels in the presence of β1-, β3- or β4-subunit. Instead, in the presence of β2a, compound 8 strongly inhibits Ca V 1.2 B15 channels over all the Ca V 1.3 splice variants tested. Given the differential distribution of β-subunits and the varied expression levels of Ca v 1.3 channel variants across various neuronal types, brain regions and organs, the use of compound 8 as a Ca V 1.3-selective antagonist needs to be further clarified. Nonetheless, the quest for discovering a highly selective and potent compound targeting Ca V 1.3 channels is a highly worthwhile goal. General synthesis information All commercially available reagents were bought from Sigma-Aldrich and Alfa Aesar, and used without further purification. Thin layer chromatography was performed using pre-coated plate (Merck silica gel 60, F254) and visualized with ultraviolet (UV) light. Flash column chromatography was carried out on Merck silica gel (230–400 mesh). 1 H and 13 C nuclear magnetic resonance (NMR) spectrums were recorded on Bruker ACF300 (300 MHz) or AMX 500 (500 MHz) spectrometer at 298 K, respectively. All J values are reported in Hz and chemical shift ( δ ) reported in p.p.m. relative to tetramethylsilane. Abbreviations for signal multiplicities are as follow: singlet (s), doublet (d), triplet (t) and multiplet (m). Mass spectra were determined by electrospray ionization (ESI) on Finnigan TSQ 7000. High-performance liquid chromatography was performed using a Shimadzu LCMS-IT-TOF system with a Phenomenex Luma C18 column (50 × 3.0 mm, 5 μm) using acetonitrile and 0.1% trifluoroacetic acid in water. The mobile phase has a flow rate of 5 ml min −1 with gradient flow of acetonitrile increasing from 5 to 90%. UV/visible detector was set at a wavelength of 254 nm. General synthetic procedure for compounds 1 , 8 and PYT Compounds 1 , 8 and PYT were synthesized according to the procedure reported by Kang. et al. [10] but with slight modifications ( Scheme 1 ). In brief, a solution of isocyanate (1 mmol) in dichloromethane (10 ml), the respective amine (1 mmol) was added and allowed to stir at room temperature overnight. The mixture was then diluted with dichloromethane (8 ml) and malonyl chloride (1.1 mmol) was added dropwise to the mixture at room temperature under vigorous stirring. Upon reaction completion (monitored by thin layer chromatography), the reaction mixture was concentrated and purified via flash column chromatography using hexane: ethyl acetate(3:1) as eluent to afford the final product. Compounds 1 , 8 and PYT were characterized via 1 H and 13 C NMR, mass spectrometry (ESI) and melting point determination ( Supplementary Figs 8,9 and 10 ). The characterization data were comparable to those reported by Kang et al. [10] Furthermore, the purity of each compound was determined by HPLC ( Supplementary Figs 11 and 12 ), and the compounds were found to have a purity value of over 98%. 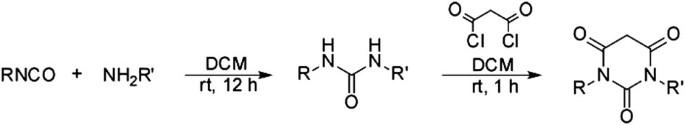Figure 7 General synthetic scheme of N,N0-disubstituted pyrimidinetrione analogue. Figure 7 General synthetic scheme of N,N0-disubstituted pyrimidinetrione analogue. Full size image 1-(4-chlorophenethyl)-3-cyclohexylpyrimidine-2,4,6(1H,3H,5H)-trione (1) White powder; 1 H NMR spectrum (CDCl 3 , 300 MHz): δ 7.21(d, J =8.4 Hz, 2H), 7.12(d, J =8.4 Hz, 2H), 4.54(m, 1H), 3.99(m, 2H) 3.55(s, 1H), 2.81(m, 2H), 2.17(m, 2H), 1.79(m, 2H), 1.58(m, 3H), 1.32(m, 3H); 13 C NMR (CDCl 3 , 75 MHz): δ 164.59, 164.41, 150.92, 136.16, 132.33, 130.13, 128.48, 55.12, 42.50, 40.02, 33.15, 28.88, 26.11, 24.93; melting point: 146.6–147.5 °C (146–148 °C; ref. 11 ); HRMS(ESI) calculated for C 18 H 21 ClN 2 O 3 [M-H] - : 347.1168; found, 347.1168. 1-(3-chlorophenethyl)-3-cyclopentylpyrimidine-2,4,6(1H, 3H, 5H)-trione (8) White solid; 1 H NMR spectrum (CDCl 3 , 500 MHz): δ 7.23-7.18(m, 3H), 7.12(d, J = 4.14 Hz, 1H), 5.12(m, 1H), 4.05(m, 2H), 3.60(s, 2H), 2.86(m, 2H), 1.92(m, 4H), 1.84(m, 2H), 1.57(m, 2H); 13 C NMR spectrum (CDCl 3 , 125 MHz): δ 164.68, 164.40, 150.79, 139.77, 134.18, 129.72, 128.96, 127.03, 126.81, 54.24, 42.48, 40.00, 33.55, 28.59, 25.42; melting point: 131.3-131.8 °C (131-132 °C; ref. 11 ); HRMS(ESI) calculated for C 17 H 19 ClN 2 O 3 [M-H] - : 333.1011; found, 333.1007. 1,3-bis(4-chlorophenethyl)pyrimidine-2,4,6(1H, 3H, 5H)-trione (PYT) White powder; 1 H NMR (CDCl 3 , 500 MHz): δ 7.28(d, J =8.15 Hz, 4H), 7.17(d, J =8.1 Hz, 4H), 4.06(t, J =7.7 Hz, 4H), 3.60(s, 2H) 2.84(t, J =7.95 Hz, 4H); 13 C NMR (CDCl 3 , 125 MHz): δ 164.18, 150.98, 136.07, 132.57, 130.23, 128.67, 42.77, 39.46, 33.26; melting point: 171.8-172.9 °C; HRMS(ESI) calculated for C 20 H 18 Cl 2 N 2 O 3 [M-H] - :403.0622; found, 403.0612. Electrophysiological recordings and data analysis Whole-cell patch-clamp electrophysiological recordings were used to characterize the recombinant rat Ca V 1.3 42 and of Ca V 1.3 42a channels [8] , and rat Ca V 1.2 B15 channel [9] . I Ca currents were recorded from transiently transfected mammalian HEK293 cells at room temperature with calcium phosphate method [16] , [17] . Outward I K currents were blocked by Cs + in the internal and external solutions. Cells were transiently transfected with the respective Ca V 1.3 and Ca V 1.2 constructs with rat β 2a -subunit and rat α 2 δ-subunit using standard calcium phosphate transfection method. For whole-cell patch-clamp recording, the internal solution (patch-pipette solution) contained the following (in mM): 138 Cs-MeSO 3 , 5 CsCl, 5.0 EGTA, 10 HEPES and 1 MgCl 2 , and 2 mg ml −1 Mg–ATP, pH 7.3 (adjusted with CsOH), and 290 mOsm with glucose. The external solution contained the following (in mM): 109 NaCl, 10 CaCl 2 , 1 MgCl 2 , 20 CsCl and 10 HEPES, (pH adjusted to 7.4 with CsOH and osmolality to 290 glucose). Pipettes of resistance 1.5–2 MΩ were used. Whole-cell currents, obtained under voltage clamp with an Axopatch 200B amplifier (Molecular Devices, Union City, CA), were filtered at 1–5 kHz and sampled at 5–50 kHz, and the series resistance was typically <5 MΩ after >80% compensation. A P/4 protocol was used to subtract on-line the leak and capacitive transients. The currents were recorded by single square pulse from holding of −70 to 10 mV for over 1 s or 100 ms with sweep interval of 20 s. Data were acquired using the software pClamp9 (Molecular Devices), and analysed and fitted using GraphPad Prism V software (San Diego, CA) and Microsoft (Seattle, WA) Excel. Data are expressed as mean values±s.e.m. Drug preparation Stock solutions were prepared by dissolving compound PYT , 1 , 8 and nimodipine (RBI) in DMSO to make a 100-mM stock solution and stored at −20 °C in the dark. Respective concentrations were freshly prepared in the bath solution from stock, and perfused (1 ml per min) into the whole recording chamber by gravity during current recording. The cell selected for patch-clamp recording were positioned as close to the outlet as possible. The external solutions were protected from light throughout the experiment. How to cite this article: Huang, H. et al. Modest Ca V 1.3 42 -selective inhibition by compound 8 is β-subunit dependent. Nat. Commun. 5:4481 doi: 10.1038/ncomms5481 (2014).